A pan-cancer proteomic perspective on The Cancer Genome Atlas Protein levels and function are poorly predicted by genomic and transcriptomic analysis of patient tumours. Therefore, direct study of the functional proteome has the potential to provide a wealth of information that complements and extends genomic, epigenomic and transcriptomic analysis in The Cancer Genome Atlas (TCGA) projects. Here we use reverse-phase protein arrays to analyse 3,467 patient samples from 11 TCGA ‘Pan-Cancer’ diseases, using 181 high-quality antibodies that target 128 total proteins and 53 post-translationally modified proteins. The resultant proteomic data are integrated with genomic and transcriptomic analyses of the same samples to identify commonalities, differences, emergent pathways and network biology within and across tumour lineages. In addition, tissue-specific signals are reduced computationally to enhance biomarker and target discovery spanning multiple tumour lineages. This integrative analysis, with an emphasis on pathways and potentially actionable proteins, provides a framework for determining the prognostic, predictive and therapeutic relevance of the functional proteome. The Cancer Genome Atlas (TCGA) is generating comprehensive molecular profiles for each of at least 33 different human tumour types ( http://cancergenome.nih.gov ). The overarching goal is to elucidate the landscape of DNA and RNA aberrations within and across tumour lineages and integrate the information with clinical characteristics, including patient outcome. Previous studies have indicated only a partial concordance between genomic copy number, RNA levels and protein levels in both patient samples and cell lines [1] , [2] , [3] at least, in part, because protein levels and, in particular, phosphoprotein levels represent an integration of the complex genomic and transcriptomic aberrations accumulated in each tumour combined with translational and post-translational regulation that cannot be fully captured by genomic and transcriptomic analysis. Hence, functional protein analysis using reverse-phase protein arrays (RPPA), which are highly applicable to study the large numbers of TCGA samples, was added to the TCGA effort to integrate proteomic characterization of tumours with already available genomic, transcriptomic and clinical information. The Clinical Proteomic Tumor Analysis Consortium (CPTAC, http://proteomics.cancer.gov/programs/cptacnetwork ) is starting to use mass spectrometry to analyse a large fraction of the human proteome for a select subset of TCGA tumours. However, a comprehensive mass spectrometry analysis across all TCGA samples is not likely to be available in the near future. Thus, while earlier TCGA analyses were primarily based on genomic and transcriptomic characteristics [4] , [5] , [6] , [7] , [8] , [9] , [10] , the current study is driven by proteomic processes within and across cancer types. Here we report an RPPA-based proteomic analysis using 181 high-quality antibodies that target total ( n =128), cleaved ( n =1), acetylated ( n =1) and phosphorylated forms ( n =51) of proteins in 3,467 TCGA patient samples across 11 ‘Pan-Cancer’ tumour types. The function space covered by the antibodies used in the RPPA analysis includes proliferation, DNA damage, polarity, vesicle function, EMT, invasiveness, hormone signalling, apoptosis, metabolism, immunological and stromal function as well as transmembrane receptors, integrin, TGFβ, LKB1/AMPK, TSC/mTOR, PI3K/Akt, Ras/MAPK, Hippo, Notch and Wnt/beta-catenin signalling. Thus, the function space encompasses major functional and signalling pathways of relevance to human cancer. The TCGA tumour types included are those with mature RPPA data: breast cancer (BRCA, n =747), colon (COAD, n =334) and rectal (READ, n =130) adenocarcinoma, renal clear cell carcinoma (KIRC, n =454), high-grade serous ovarian cystadenocarcinoma (OVCA, n =412), uterine corpus endometrial carcinoma (UCEC, n =404), lung adenocarcinoma (LUAD, n =237), head and neck squamous cell carcinoma (HNSC, n =212), lung squamous cell carcinoma (LUSC, n =195), bladder urothelial carcinoma (BLCA, n =127) and glioblastoma multiforme (GBM, n =215) [4] , [5] , [6] , [7] , [8] , [9] , [10] . We show that the functional proteome gives important, independent insights into TCGA data that are not captured by genomics or transcriptomics. Although samples predominantly cluster by tumour lineage, we also show that part of the tissue dominant effects can be removed computationally to elucidate common processes driving cellular behaviour across tumour lineages. We present proteins and pathways that correlate with outcomes within certain tumour lineages and we identify multiple protein links and proteins that are associated with pathway activation. Taken together, the data and analytical resources presented in this manuscript are aimed at facilitating future research for targeted therapies that span multiple tumours. Correlations between protein and other data types Protein data for 3,467 samples across 11 diseases were compared with mRNA, miRNA, copy number and mutation data for the same samples. A novel approach, called ‘replicates-based normalization’ (RBN, Methods), mitigated batch effects facilitating creation of a single Pan-Cancer protein data set merging samples across six different batches. The RBN output is equivalent to all 3,467 samples being run in a single batch. In contrast to random ( trans ) protein:mRNA pairs (mean Spearman’s ρ =−0.006), almost half of matched ( cis ) protein:mRNA pairs in the RBN set demonstrated correlation beyond that expected by chance (mean Spearman’s ρ =0.3) in both the overall Pan-Cancer data set ( t-test P <2.2e−16 , n =206 matched protein:mRNA pairs) and within particular diseases ( Fig. 1a , Supplementary Fig. 1 , Supplementary Data 1,2 ). Approximately 44% of matched ( cis ) protein:mRNA pairs had a correlation >=0.3. For micro-RNAs, as expected, ( trans ) protein:miRNA correlations were much weaker with a mean positive Spearman’s ρ =0.07 and a mean negative Spearman’s ρ =−0.07 ( Supplementary Data 3 ). In contrast, ( trans ) protein:protein correlations, including phosphoproteins, were higher (mean positive Spearman’s ρ =0.15, mean negative Spearman’s ρ =−0.13, Supplementary Data 4 ). Detailed protein:protein and phosphoprotein:protein correlations across the total data set and in particular diseases are available at the TCPA portal [11] . The results show, not surprisingly, that matched ( cis ) mRNA:protein correlations were the highest on average ( ρ =0.3), followed by ( trans ) protein:protein correlations ( ρ ≈±0.15), whereas ( trans ) protein:miRNA correlations were lowest on average ( ρ =±0.07). 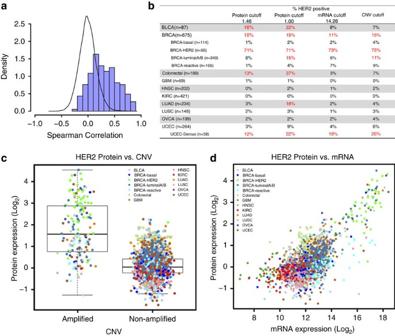Figure 1: HER2 RPPA correlations with copy number and mRNA. (a) Histogram of Spearman’s rank correlation (ρ-values) for 206 pairs of proteins and matched mRNAs across all tumour types. The black curve represents the background ofρvalues using 28,960 random protein-mRNA pairs in the same data set. (b) Crosstab identifyingHER2-positive tumours by copy number, mRNA expression and protein expression across 11 tumour types. Cutoffs are defined in Methods. BRCA and UCEC are subdivided for clinical relevance regarding HER2 protein levels. Total sample numbers with analyses for all three platforms (CNV, mRNA and protein) are indicated in parentheses. Percentages ≥10% are highlighted (red). (c) Relationship betweenHER2copy number and HER2 protein level by RPPA across all tumour types (n=2,479). The box represents the lower quartile, median and upper quartile, whereas the whiskers represent the most extreme data point within 1.5 × inter-quartile range from the edge of the box. Each point represents a sample, colour coded by tumour type or subtype. As expected,HER2amplified samples have much higher HER2 protein levels than non-amplified samples. (d) Relationship betweenHER2mRNA and protein expression across all tumour types (n=2,479). Each protein represents a sample, colour coded by tumour type or subtype. Spearman’s correlation between HER2 protein and mRNA is 0.53. Figure 1: HER2 RPPA correlations with copy number and mRNA. ( a ) Histogram of Spearman’s rank correlation ( ρ -values) for 206 pairs of proteins and matched mRNAs across all tumour types. The black curve represents the background of ρ values using 28,960 random protein-mRNA pairs in the same data set. ( b ) Crosstab identifying HER2 -positive tumours by copy number, mRNA expression and protein expression across 11 tumour types. Cutoffs are defined in Methods. BRCA and UCEC are subdivided for clinical relevance regarding HER2 protein levels. Total sample numbers with analyses for all three platforms (CNV, mRNA and protein) are indicated in parentheses. Percentages ≥10% are highlighted (red). ( c ) Relationship between HER2 copy number and HER2 protein level by RPPA across all tumour types ( n =2,479). The box represents the lower quartile, median and upper quartile, whereas the whiskers represent the most extreme data point within 1.5 × inter-quartile range from the edge of the box. Each point represents a sample, colour coded by tumour type or subtype. As expected, HER2 amplified samples have much higher HER2 protein levels than non-amplified samples. ( d ) Relationship between HER2 mRNA and protein expression across all tumour types ( n =2,479). Each protein represents a sample, colour coded by tumour type or subtype. Spearman’s correlation between HER2 protein and mRNA is 0.53. Full size image A similar analysis for CNV versus protein fold change showed a mean fold change of 1.05 for amplifications and 0.95 for deletions in cis ( Supplementary Data 5,6 ). Mutation versus protein ( cis ) analysis showed a mean fold change of 1.2 for mutations that increased expression, and 0.9 for mutations that decreased expression ( Supplementary Data 7,8 ), showing that mutations, in general, are associated with greater average fold changes than copy-number variations, perhaps due to nonsense-mediated RNA degradation. Complete tables are available at: ( http://bioinformatics.mdanderson.org/main/TCGA/Pancan11/RPPA ). HER2 analysis as an example We then focused on HER2 as an illustrative example. A comparison of relative HER2 ( ERBB2 ) protein levels across tumour types illustrates the potential utility of a pan-cancer proteomic analysis. While the overall HER2 protein:mRNA correlation was 0.53 ( P= 5e−177), the correlation was 0.61 (P= 1e−69) in BRCA, where HER2-targeted therapy has been demonstrated to be effective (Spearman’s correlations Fig. 1 , Supplementary Data 1 ). Importantly, phosphoHER2Y1248 protein:mRNA correlation was 0.552 (P= 3e−54) and HER2:phosphoHER2Y1248 protein:protein correlation was 0.67 (P= 4e−98) in breast cancer consistent with ability of RPPA to capture both total and phosphoprotein levels from TCGA samples ( n =2,503 for overall and n =674 for BRCA correlations and P -value computations using t -distribution test and adjusted for multiple hypotheses testing using Benjamini Hochberg adjustment. n =2,479 in Fig. 1 ). On the basis of correlations with DNA, RNA and protein levels in HER2 -positive breast cancers, HER2 protein levels were defined as elevated if the relative HER2 level was ≥1.46 (see Methods) ( Fig. 1b–d ). We also set a cutoff at the relative protein level of 1.00 (which is approximately equivalent to 3+ staining on clinical immunohistochemistry analysis of the breast cancer samples and represent the top 12% of patient samples, see Methods). Using either cutoff, 10–15% of breast cancers demonstrated elevated HER2 by DNA copy number, RNA and protein consistent with clinical data [12] , [13] ( Fig. 1b ). On the basis of those cutoffs, approximately 25% of serous endometrial cancers had coordinated elevation of HER2 DNA, RNA and protein levels, an even higher frequency than breast cancer. BLCA, colorectal cancer and LUAD demonstrated a higher frequency of elevated protein levels than predicted by mRNA and DNA levels. In an independent cohort of 26 LUAD cell lines using the same cutoffs, seven of the cell lines had high HER2 protein levels, whereas only two cell lines had high mRNA levels, consistent with our observation of elevated protein levels occurring at a higher frequency than elevated RNA levels ( Supplementary Table 1 , Supplementary Fig. 2 ) [14] . Discordance between HER2 DNA copy number and protein levels has been observed in multiple individual tumour types previously [15] , [16] , [17] , [18] , [19] , [20] . Besides diversity in methodology, a number of cancer-specific hypotheses including post-translational regulation of HER2 expression, cytoplasmic HER2 localization [16] , intratumoral heterogeneity of HER2 amplification [19] or polysomy 17 (refs 17 , 20 ) have been suggested. This clearly contrasts breast cancer, where HER2 levels are usually highly correlated at the DNA, RNA and protein level [21] , [22] , [23] , [24] . With the advent of TDM1 toxin conjugate therapy (trastuzumab emtansine) [25] , [26] , the higher frequency of elevated HER2 protein levels in BLCA, LUAD, endometrial and colorectal cancers supports the (pre)clinical exploration of TDM1, which binds HER2 to deliver a potent cell-cycle toxin (a mechanism of activity independent from trastuzumab, a drug with limited activity in endometrial cancer in previous studies [27] ) in these tumour lineages. Unsupervised clustering analysis Unsupervised clustering identified eight robust clusters (Clusters A-H, Fig. 2a ) when batch effects were mitigated by RBN. Not surprisingly, RBN cluster membership is defined primarily by tumour type with the exception of cluster_E and cluster_F, which include multiple diseases ( Fig. 2b ). Bladder cancer, however, did not generate a dominant cluster but, rather, was co-located with other tumour lineages in multiple clusters. To identify potential discriminators of clusters, we compared the ability of proteins, RNAs, miRNAs and mutations for each cluster to different samples from those in all other clusters (top 25 discriminators, Supplementary Tables 2–5 , all the discriminators at http://bioinformatics.mdanderson.org/main/TCGA/Pancan11/RPPA ). 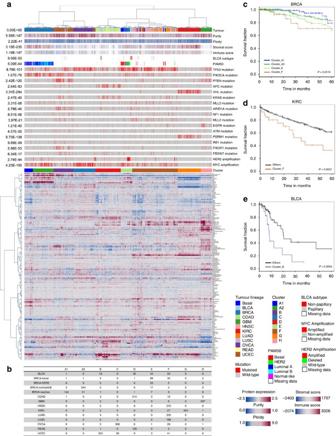Figure 2: Unsupervised clustering and analyses based on the RBN data set. (a) Heatmap depicting protein levels after unsupervised hierarchical clustering of the RBN data set consisting of 3,467 cancer samples across 11 tumour types and 181 antibodies. Protein levels are indicated on a low-to-high scale (blue-white-red). Eight clusters are defined. Cluster_A has been subdivided into two clusters (A1 and A2), based on the differences between BRCA reactive and remaining luminal subtypes5. Annotation bars include tumour type (BRCA-basal separately indicated); purity and ploidy (ABSOLUTE algorithm); stromal and immune scores (ESTIMATE algorithm); BRCA (PAM50 classification) and BLCA subtype; 16 significantly mutated genes and two frequently observed amplifications. The statistical significance of correlations between the clusters and each variable is indicated to the left of each annotation bar (n=3,467,χ2-test, Fisher’s Exact and ANOVA’s F test. See Methods). (b) Crosstab showing the number of tumour samples in each cluster. (c–e) Kaplan–Meier curves showing overall survival of (c) the BRCA located in four separate clusters (A1, A2, E and F,n=740), (d) KIRC in cluster_F versus KIRC in other clusters (n=454) and (e) BLCA in cluster_B versus BLCA in other clusters (n=127). Follow-up was capped at 60 months due to limited number of events beyond this time. Statistical difference in outcome between groups is indicated byP-value (log-rank test). A high-resolution, interactive version of the heatmap with zooming capability, can be found at (http://bioinformatics.mdanderson.org/main/TCGA/Pancan11/RPPA). Supplementary Table 2 highlights the contribution of individual proteins in driving the different clusters. Associations of specific mutations and copy-number changes with the clusters were primarily based on known associations of mutations and copy-number changes with tumour lineage [4] , [5] , [6] , [7] , [8] , [9] , [10] . Figure 2: Unsupervised clustering and analyses based on the RBN data set. ( a ) Heatmap depicting protein levels after unsupervised hierarchical clustering of the RBN data set consisting of 3,467 cancer samples across 11 tumour types and 181 antibodies. Protein levels are indicated on a low-to-high scale (blue-white-red). Eight clusters are defined. Cluster_A has been subdivided into two clusters (A1 and A2), based on the differences between BRCA reactive and remaining luminal subtypes [5] . Annotation bars include tumour type (BRCA-basal separately indicated); purity and ploidy (ABSOLUTE algorithm); stromal and immune scores (ESTIMATE algorithm); BRCA (PAM50 classification) and BLCA subtype; 16 significantly mutated genes and two frequently observed amplifications. The statistical significance of correlations between the clusters and each variable is indicated to the left of each annotation bar ( n =3,467, χ 2 -test, Fisher’s Exact and ANOVA’s F test. See Methods). ( b ) Crosstab showing the number of tumour samples in each cluster. ( c – e ) Kaplan–Meier curves showing overall survival of ( c ) the BRCA located in four separate clusters (A1, A2, E and F, n =740), ( d ) KIRC in cluster_F versus KIRC in other clusters ( n =454) and ( e ) BLCA in cluster_B versus BLCA in other clusters ( n =127). Follow-up was capped at 60 months due to limited number of events beyond this time. Statistical difference in outcome between groups is indicated by P -value (log-rank test). A high-resolution, interactive version of the heatmap with zooming capability, can be found at ( http://bioinformatics.mdanderson.org/main/TCGA/Pancan11/RPPA ). Full size image Cluster_E includes 70% of basal-like breast cancers, the majority of HER2-positive breast cancers (87%) and the largest group of bladder cancers (35%), including many with amplified HER2 ( Fig. 2a,b ). Cluster_E is defined by TP53 mutations, elevated HER2, cyclinB1 and Rab25 protein levels and low ER and PR levels ( Supplementary Table 2 ). Cluster_F includes smoking-related, upper aerodigestive tract cancers (HNSC, LUAD and LUSC) and subsets of other tumour types. Cluster_F contains the majority of a ‘squamous cancer’ subset (94%), P <0.0001, χ 2 -test), recently identified through other Pan-Cancer subtype analyses [28] . However, cluster_F also contains an equally large number of non-squamous tumours, predominantly LUAD (58% of the non-squamous tumours in cluster_F). Membership in cluster_F is associated with TP53 mutations and elevated total and phosphorylated EGFR (EGFRp1068 and EGFRp1173), phosphorylated SRC (SRCpY527) and low ER and PR levels. Although TP53 mutations are usually associated with copy-number changes and a limited number of recurrent mutations in cancer genes [7] , cluster_F is unexpectedly enriched in recurrent cancer gene mutations ( Supplementary Table 6 ). Within the group of current smokers in cluster_F ( Supplementary Fig. 3 ), tumours with TP53 mutations show significantly higher rates of co-mutations in the top-25 driver mutations (Methods, P <0.0001, t -test, n =162). 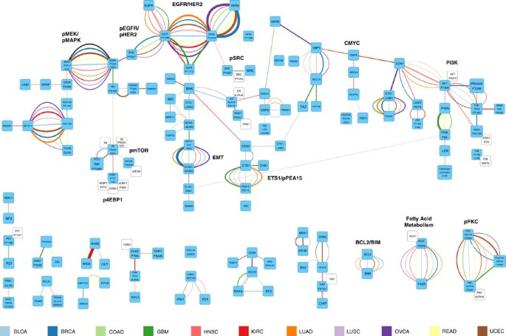Figure 6: Unbiased data-driven signalling network. Unbiased signalling network based on a probabilistic graphical model analysis, visualizing all 11 tumour lineages individually. Interplay between nodes was quantified using scores from the graphical model analysis (see Methods) that identify links between nodes whilst controlling for the effects of all other observed nodes. The strength of links is indicated by the thickness of the line while the colour indicates the tumour lineage in which the link was observed; only the strongest links are shown. Nodes in white are related nodes that were highly correlated and therefore merged before network analysis. The adjacent correlated (green) node was then used for network generation. Positive (negative) correlations are indicated with continuous (dotted) lines. A high-resolution image of the network can be found online (http://bioinformatics.mdanderson.org/main/TCGA/Pancan11/RPPA). Hormonally responsive ‘women’s cancers’ (luminal BRCA, OVCA, UCEC) form a major tumour super cluster. Basal-like breast cancers and HER2 -positive breast cancers are distinct from luminal breast cancers, being located in cluster_E (the majority of HER2 (87%) and basal-like (70%)) and cluster_F (subset of basal-like (25%)). This is consistent with previous data suggesting that HER2 and basal-like breast cancer are distinct from luminal breast cancer [5] . In light of the recent identification of a ‘reactive’ breast cancer subtype [5] , we split the luminal cluster into two (reactive breast cluster_A1 and non-reactive ER-positive breast cluster_A2). For some tumour lineages, localization to different clusters reflects differences in prognosis. Breast cancers located in different clusters demonstrate distinct outcomes: tumours in cluster_E and cluster_F are associated with the worst outcome, probably due to the inclusion of HER2 -positive and basal-like tumours. Reactive cluster_A1 shows a better outcome than cluster_A2 ( Fig. 2c ). The poor outcome associated with KIRC in cluster_F ( Fig. 2d ) may be due to the absence of VHL mutations (Fisher’s exact test (FE), P =0.008, n =454), which has been associated with a worse outcome in kidney cancer [29] . Bladder cancers in cluster_B show worse survival compared with all other BLCA, which may be due to associations with TP53 mutation (FE, P <0.001) and cMYC amplification (FE, P =0.042) ( n =127) ( Fig. 2e ). We evaluated the concordance between RBN protein clusters and mRNA clusters derived from the same sample set ( Supplementary Table 7 ). Most of the protein clusters predominantly corresponded to a single respective mRNA cluster despite the mRNA clusters being defined with a pool of about 20,000 mRNAs, whereas only 181 proteins and phosphoproteins were used to generate the protein clusters. Therefore, many of the features defining the mRNA clusters were captured by just a few proteins. This agreement between RNA- and protein-based clustering provides validation of the quality of the protein data, as well as the selection of protein targets in the arrays. However, clusters E and F were noticeably different from their mRNA counterparts. Unlike protein cluster_E that contains BLCA and BRCA, bladder cancer formed a separate cluster in mRNA data, distinct from HER2 and basal-like breast cancers. LUAD also formed a separate mRNA cluster, distinct from the LUSC/HNSC mRNA cluster, unlike protein cluster_F that contains LUAD as well as LUSC and HNSC. Reduction of tissue-specific proteomic signatures Tumour lineage represents the dominant determinant of protein clustering using the RBN approach ( Fig. 2 ). We, therefore, investigated whether further transforming the RBN data to reduce tissue signatures by median centering within tissue types (MC, see Methods) would identify clinically or biologically relevant protein patterns that span multiple tumour lineages ( Fig. 3a ). Using MC, we obtained seven clusters (I-VII) that were no longer strongly correlated with tumour lineage, as evident from the top annotation bar in Fig. 3a ( Supplementary Fig. 4 ), and from the tissue versus cluster cross-tabulation ( Fig. 3b ). This allowed exploration of molecular events that spanned multiple tissues, which was not possible with the RBN approach. Supplementary Table 8 shows a contingency table with the distribution of samples across RBN versus MC clusters, highlighting the differences between the clusters. 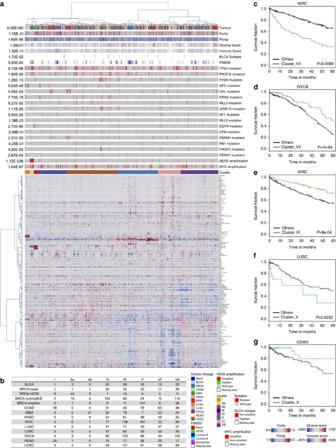Supplementary Tables 9–12 show the top 25 proteins, mRNAs, miRNAs and mutations that discriminated different MC clusters (full table available at http://bioinformatics.mdanderson.org/main/TCGA/Pancan11/RPPA ). Figure 3: Unsupervised clustering and analyses based on the MC data set. (a) Heatmap showing protein expression after unsupervised hierarchical clustering of 3,467 cancer samples across 11 tumour types and 181 antibodies. Protein levels are indicated on a low-to-high scale (blue-white-red). Seven clusters were defined. Cluster_II has been subdivided manually into two clusters (IIa and IIb) based on significant difference in expression of the proteins of interest (HER2 and EGFR). Annotation bars include tumour lineage (BRCA-basal separately indicated), purity and ploidy (ABSOLUTE algorithm); stromal and immune scores (ESTIMATE algorithm); BRCA (PAM50 classification) and BLCA subtype; 16 significantly mutated genes and two frequently observed amplifications. Statistical significance of the correlations between the clusters and each variable is indicated left of the annotation bars (n=3,467,χ2-test, Fisher’s Exact, and ANOVA’s F test. See Methods). (b) Crosstab showing the number of tumour samples in each cluster. (c–g) Kaplan–Meier curves showing overall survival in (c) the KIRC in cluster_VII versus in all other clusters (n=454), (d) OVCA in cluster_VII versus in all other clusters (n=412), (e) KIRC in cluster_IV versus in all other clusters (n=454), (f) LUSC in cluster_V versus in all other clusters (n=195) and (g) COAD in cluster_V versus in all other clusters (n=334). Follow-up has been capped at 60 months months, due to limited number of events beyond this time. Statistical difference in outcome between groups is indicated byP-value (log-rank test). A high-resolution, interactive version of the heatmap with zooming capability, can be found at (http://bioinformatics.mdanderson.org/main/TCGA/Pancan11/RPPA). Figure 3: Unsupervised clustering and analyses based on the MC data set. ( a ) Heatmap showing protein expression after unsupervised hierarchical clustering of 3,467 cancer samples across 11 tumour types and 181 antibodies. Protein levels are indicated on a low-to-high scale (blue-white-red). Seven clusters were defined. Cluster_II has been subdivided manually into two clusters (IIa and IIb) based on significant difference in expression of the proteins of interest (HER2 and EGFR). Annotation bars include tumour lineage (BRCA-basal separately indicated), purity and ploidy (ABSOLUTE algorithm); stromal and immune scores (ESTIMATE algorithm); BRCA (PAM50 classification) and BLCA subtype; 16 significantly mutated genes and two frequently observed amplifications. Statistical significance of the correlations between the clusters and each variable is indicated left of the annotation bars ( n =3,467, χ 2 -test, Fisher’s Exact, and ANOVA’s F test. See Methods). ( b ) Crosstab showing the number of tumour samples in each cluster. ( c – g ) Kaplan–Meier curves showing overall survival in ( c ) the KIRC in cluster_VII versus in all other clusters ( n =454), ( d ) OVCA in cluster_VII versus in all other clusters ( n =412), ( e ) KIRC in cluster_IV versus in all other clusters ( n =454), ( f ) LUSC in cluster_V versus in all other clusters ( n =195) and ( g ) COAD in cluster_V versus in all other clusters ( n =334). Follow-up has been capped at 60 months months, due to limited number of events beyond this time. Statistical difference in outcome between groups is indicated by P -value (log-rank test). A high-resolution, interactive version of the heatmap with zooming capability, can be found at ( http://bioinformatics.mdanderson.org/main/TCGA/Pancan11/RPPA ). Full size image Cluster_I was primarily driven by phosphoPEA15, YB1, EEF2 and ETS1 proteins ( Supplementary Table 9 ), which were markedly elevated in a subset of colorectal tumours (18%). Cluster_I exhibited enrichment of APC and KRAS mutations, very few HER2 amplifications, but moderately high HER2 protein levels ( Fig. 3a , Supplementary Tables 9,12 ). It also had evidence for suppressed DNA damage response, apoptosis, and mTOR and MAPK pathway levels ( Fig. 4b ). Cluster_II was divided into two further subclusters, one primarily driven by HER2 (IIa) and one by EGFR (IIb) ( Supplementary Table 9 ). Interestingly, a subset of OVCA, UCEC, BLCA and LUAD samples that had HER2 amplification and HER2 protein levels comparable to breast HER2+ samples were located in cluster_IIa, raising intriguing opportunities for (pre)clinical investigation of HER2 targeted therapy and particularly TDM1 therapy as noted above. Cluster_IIa also had activated RTK and cell cycle pathways, but suppressed hormonal signalling pathways ( Fig. 4b ). Similarly, a subset of HNSC and lung samples that had EGFR levels comparable to a subset of GBM samples (28%) was located in cluster_IIb, warranting exploration of potential benefit from EGFR pathway-targeted drugs [30] . Tumours in cluster_IIb were enriched in EGFR mutations, contained few PTEN mutations, and had elevated RTK pathway and suppressed mTOR pathway signatures. Clusters III-VII consisted of a mixture of all tissue types. Cluster_V was the most distinctive, exhibiting a strong ‘reactive’ signature [5] , with elevated MYH11, RICTOR, Caveolin1 and Collagen VI, and an activated EMT signature. Cluster_V also exhibited low cell cycle, Wnt-signalling and DNA damage response pathway signatures. Cluster_V contained the majority of the breast reactive samples along with multiple other tumours with a ‘reactive’ signature consistent with the reactive phenotype being a pan-cancer characteristic. Cluster_III was the antithesis of ‘reactive’ cluster_V and was primarily driven by elevated BRAF, ER-alpha and E-cadherin ( Fig. 3a ). In contrast to cluster_V, cluster_III had low EMT, apoptosis and MAPK pathway signatures, but high DNA damage and hormonal pathway signatures. Patients in cluster_III may potentially benefit from (pre)clinical hormone targeting therapies. Cluster_III also had high beta-catenin levels, suggesting activation of the canonical Wnt-signalling pathway. Cluster_IV also had high beta-catenin, as well as activated AKT, MAPK and mTOR pathways, but suppressed DNA damage, apoptosis, EMT and cell cycle pathways. Cluster_IV and cluster_VII were antitheses. The high levels of phosphoAKT and phosphoMAPK in cluster_IV, suggested evaluation of (pre)clinical benefit from kinase-targeted therapies. Cluster_VI showed high EMT, cell cycle, apoptosis, mTOR and MAPK pathway signatures, also suggesting further evaluation of kinase-targeted therapies. Cluster_VI had low beta-catenin, consistent with suppressed Wnt-signalling. 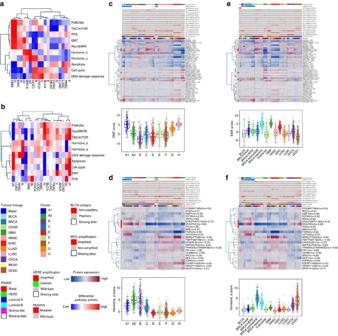Cluster_VII also showed low beta-catenin, with suppressed AKT, MAPK, mTOR and RTK pathways. Figure 4: Pathway analyses. Pathway analyses of the data set by RBN clusters, MC clusters and tumour type. For pathway predictor members seeSupplementary Table 13. (a,b) Heatmaps depicting mean pathway scores after unsupervised hierarchical clustering on tumour lineages and protein clusters based on the (a) RBN and (b) MC data sets. The heatmaps were clustered on both axes. As expected, RBN clusters show a strong association with tumour lineages, with very similar patterns between them, whereas MC clusters do not associate with any particular tumour lineage. (c–f) The heatmaps, supervised on the sample axis, depict the protein levels of the pathway members and of proteins with a high correlation (ρ>0.3/ρ<−0.3, Spearman’s correlation) to the pathway predictor across RBN clusters (c,d) and tumour lineages (e,f). The EMT pathway (c,e) and the hormone_a pathway (d,f) are shown. Samples are first sorted by either cluster (c,d) or tumour lineage (e,f), then by pathway score (from low to high) within cluster or tumour lineage. Dotplots (lower panel) represent the pathway score for each sample. Each box represents the lower quartile, median and upper quartile, whereas the whiskers represent the most extreme data point within 1.5 × inter-quartile range from the edge of the box. Annotation bars (selected fromFig. 2) are included if statistically associated with the pathway score (P<0.05, Kruskal–Wallis test,n=3,467). Pathway members are marked in red on the left hand side. High-resolution images of the heatmaps can be found online (http://bioinformatics.mdanderson.org/main/TCGA/Pancan11/RPPA). Figure 4: Pathway analyses. Pathway analyses of the data set by RBN clusters, MC clusters and tumour type. For pathway predictor members see Supplementary Table 13 . ( a , b ) Heatmaps depicting mean pathway scores after unsupervised hierarchical clustering on tumour lineages and protein clusters based on the ( a ) RBN and ( b ) MC data sets. The heatmaps were clustered on both axes. As expected, RBN clusters show a strong association with tumour lineages, with very similar patterns between them, whereas MC clusters do not associate with any particular tumour lineage. ( c – f ) The heatmaps, supervised on the sample axis, depict the protein levels of the pathway members and of proteins with a high correlation ( ρ >0.3/ ρ <−0.3, Spearman’s correlation) to the pathway predictor across RBN clusters ( c , d ) and tumour lineages ( e , f ). The EMT pathway ( c , e ) and the hormone_a pathway ( d , f ) are shown. Samples are first sorted by either cluster ( c , d ) or tumour lineage ( e , f ), then by pathway score (from low to high) within cluster or tumour lineage. Dotplots (lower panel) represent the pathway score for each sample. Each box represents the lower quartile, median and upper quartile, whereas the whiskers represent the most extreme data point within 1.5 × inter-quartile range from the edge of the box. Annotation bars (selected from Fig. 2 ) are included if statistically associated with the pathway score ( P <0.05, Kruskal–Wallis test, n =3,467). Pathway members are marked in red on the left hand side. High-resolution images of the heatmaps can be found online ( http://bioinformatics.mdanderson.org/main/TCGA/Pancan11/RPPA ). Full size image Interestingly, clinical outcomes correlated with MC cluster membership, indicating the power to identify important tissue-independent processes. COAD in cluster_V had better outcome compared with COAD located in other clusters ( Fig. 3g ) ( n =334), which may, in part, be due to depletion of mutations in TP53 (6 versus 15%, Fisher’s Exact (FE) P =0.05), APC (14 versus 25%, FE P =0.044) and KRAS (5 versus 16%, FE P =0.013), consistent with previous literature showing these are associated with a worse outcome [31] , [32] , [33] . The poor outcome for KIRC in cluster_VII may be partly due to enrichment of TP53 mutations (6 versus 0.8%, FE P =0.005, n =454) ( Fig. 3c ). In contrast, KIRC in cluster_IV are associated with better prognosis ( Fig. 3e ). For OVCA, membership in cluster_VII is associated with improved survival ( Fig. 3d ). LUSC in cluster_V appear to have worse prognosis, which may be related to elevated EMT pathway activity compared with LUSC in other clusters ( Supplementary Fig. 5 ) [34] , [35] , as well as low E-cadherin protein levels ( Fig. 3f ). Thus, reduction of tissue-specific signatures reveals a number of processes that transcend tissue boundaries and may represent cross-tissue biological, prognostic and therapeutic opportunities. Analysis of pathways and targets To capitalize on the RPPA data, we developed a series of pathway predictors (see Methods), based on member proteins selected by literature review ( Supplementary Table 13 ). TSC/mTOR signalling, which integrates information from the PI3K/Akt, Ras/MAPK and LKB1/AMPK pathways [36] , was treated as a separate pathway, as was the hormone_a (ER, pER and PR) and a series of downstream components of the hormone signalling pathway (hormone_b [37] , [38] , [39] ). All proteins and genomic events with a Spearman’s ρ >0.3 or ρ <−0.3 for association with the pathway score are also presented (See methods, Fig. 4 , Supplementary Figs 6–9 , Supplementary Table 13 ) providing additional information on potential pathway membership. In general in the RBN analysis, pathway scores were associated with tumour lineage ( Fig. 4a , Supplementary Fig. 10 ). In Figure 4a,b , each cell in the heatmap represents the mean pathway score for that cluster or tumour lineage. Blue represents a suppressed pathway, red means an activated pathway and white represents a score that does not differ across the set (see Methods). As expected, individual RBN clusters ( Fig. 4a ) show similar pathway scores to their dominant constituent tumour lineages, for example, GBM is similar to cluster_H, KIRC is similar to cluster_G, etc. However, as clusters E and F do not consist of a single predominant lineage, their pathway score pattern is not concordant with any one tumour lineage. Similarly, the MC heatmap ( Fig. 4b ) shows that MC clusters, in which tissue specific effects are removed, do not reflect a single tumour type. This emergent phenotype illustrates the mitigation of tissue-specific signatures by MC, and the emergence of new, pan-cancer patterns that span multiple tumour types. In Supplementary Fig. 10 , the data are transformed so that the colour spectrum in the heatmaps represents absolute values of pathway scores (where only score magnitude is considered) and thus reflects ‘distance from the global pathway mean’, rather than relative protein level (see Methods). This emphasizes that both low (for example, inhibitors) and high protein levels can be markers of pathway activity. Thus in Supplementary Fig. 10 , UCEC and HNSC have a near identical hormone_a score, caused by a high (UCEC) and low (HNSC) protein score, respectively. The pathway-based analyses benefit hugely from the large data set providing sufficient power to identify associations that could otherwise not be robustly identified. Focusing on individual pathway analysis ( Fig. 4c–f , Supplementary Figs 6–9 ), the high degree of correlation between pathway members, including phosphoproteins, supports the ability of RPPA to capture high-quality information including phosphoprotein levels from TCGA samples. Unexpectedly, the proteins driving the pathway signatures varied across individual tumours and tumour lineages, as did the associated proteins and genomic aberrations ( Fig. 4 , Supplementary Figs 6,8 ). This suggests that intrinsic gene expression patterns or mutational patterns provide important contributions to convergent functional pathway output. The EMT signature, which may also represent reactive stroma, showed the greatest variation, being markedly elevated in GBM and reactive BRCA tumours ( Fig. 4c,e ). Significant variation in EMT was also observed within disease type and RBN clusters. For example, Cluster_F (HNSC, LUAD, LUSC) showed a separation into distinct epithelial and mesenchymal groups based on the EMT score and related protein EMT markers. RTK and downstream signalling signatures were elevated in GBM, likely due to EGFR amplification and activation of downstream signalling events ( Fig. 2 ). Endometrial, ovarian and most breast cancers demonstrated a high hormone_a signature ( Fig. 4d,f ). However, an elevated hormone_b signature, indicative of functional downstream activation, was restricted to luminal, reactive and HER2-positive breast cancers ( Supplementary Fig. 11 ) suggesting differential ‘wiring’ of hormonal signalling across tumour lineages. HER2-positive breast cancers, whether ER-positive or -negative, demonstrated elevated levels of GATA3, INPP4B and AR (hormone_b signature) suggestive of active downstream hormonal signalling despite low levels of ER, pER and PR in many of the HER2-positive tumours ( Fig. 2 , Supplementary Fig. 11 ). A subset of endometrial cancers had massively elevated pAkt levels, likely due to the high frequency of coordinated genomic aberrations in the PI3K pathway, in particular, the loss/mutation of PTEN [10] , [40] , which is consistent with responsiveness of endometrial cancers to PI3K pathway inhibitors [41] , [42] . We analysed a number of potentially actionable proteins ( n =25, Fig. 5a,b ), selected based on a literature review ( Supplementary Methods ) for associations with proteomic and genomic events as well as for potential ability of proteomics to identify patients likely to benefit from targeted therapies. Luminal breast cancers (including AR-positive triple-negative breast cancers that cluster with luminal breast cancers) demonstrated selective elevation of AR, BCL2, FASN and pACC, suggesting these molecules or their associated pathways as potential therapeutic targets. The elevation of HER3 in KIRC may represent a therapeutic opportunity. SRC is activated in all but the hormone-responsive and bladder cancers, offering another potential therapeutic opportunity. EGFR activity, in general, parallels SRC activity, but in GBM is associated with NOTCH1 and HER3 activation, suggesting an interesting opportunity for exploration of combination therapy in (pre)clinical studies. PhosphoSRC, which is a downstream target of EGFR, was highly expressed in a subset of HNSC tumours, suggesting that these may be more sensitive to EGFR targeting strategies. As noted above, HER2 levels are elevated in a subset of UCEC, BLCA, BRCA and colorectal cancers and may represent responsiveness to HER2-targeted therapy. 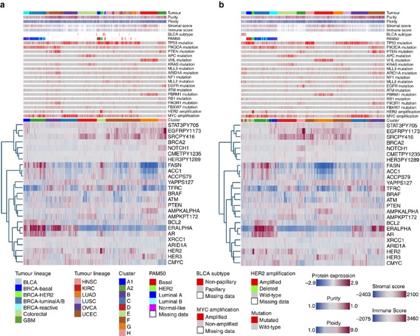MYC, which may become targetable by emerging therapeutic approaches [43] , is selectively amplified and expressed in high-grade serous ovarian cancer and may represent an important target in this disease that currently lacks targeted opportunities [7] . Figure 5: Analyses of selected potentially actionable proteins. (a,b) Heatmaps, supervised on the sample axis, depicting protein level of 25 proteins that are (potentially) actionable based on the RBN data set. Proteins were ordered by unsupervised hierarchical clustering and samples were ordered by (a) cluster and (b) tumour lineage membership and within each ordered by unsupervised hierarchical clustering. Annotation bars include tumour lineage, purity and ploidy (ABSOLUTE algorithm); stromal and immune scores (ESTIMATE algorithm); BRCA (PAM50 classification) and BLCA subtype; 16 significantly mutated genes and two frequently observed amplifications. High-resolution images of the heatmaps can be found online (http://bioinformatics.mdanderson.org/main/TCGA/Pancan11/RPPA). Figure 5: Analyses of selected potentially actionable proteins. ( a , b ) Heatmaps, supervised on the sample axis, depicting protein level of 25 proteins that are (potentially) actionable based on the RBN data set. Proteins were ordered by unsupervised hierarchical clustering and samples were ordered by ( a ) cluster and ( b ) tumour lineage membership and within each ordered by unsupervised hierarchical clustering. Annotation bars include tumour lineage, purity and ploidy (ABSOLUTE algorithm); stromal and immune scores (ESTIMATE algorithm); BRCA (PAM50 classification) and BLCA subtype; 16 significantly mutated genes and two frequently observed amplifications. High-resolution images of the heatmaps can be found online ( http://bioinformatics.mdanderson.org/main/TCGA/Pancan11/RPPA ). Full size image To determine whether protein levels, including phosphoproteins, can predict patient outcome, we determined correlations with overall survival (see TCPA) [11] for a comprehensive analysis) using Cox Proportional Hazards (CoxPH) models. In the complete Pan-Cancer data set, 80 (including 24 phosphoproteins) of the 181 proteins demonstrated a significant (corrected for multiple comparisons) correlation with outcome. Importantly, 57 proteins, including 19 phosphoproteins, showed a multiple comparison corrected correlation with outcome in KIRC. However, with the exception of breast cancer (13 candidates), this approach showed five or fewer proteins correlating with outcome in other tumour lineages. Why kidney cancer shows such strong correlations is not completely understood, but may reflect the maturity of the outcome data in this data set [44] . For some of the other diseases included in the Pan-Cancer data set, the associated outcome data are immature, for example, the low number of events in the BRCA and endometrial cancer data sets limits the ability to detect the prognostic and predictive value of protein markers. To extend the single-protein analysis available in TCPA, we performed a formal training/test set analysis of pathways and potentially actionable proteins. As indicated in Supplementary Table 14 , 17 predictors (four pathways, nine total proteins and four phosphoproteins) passed a rigorous training/test set approach and showed a robust correlation with outcome in at least one disease. As expected from the analysis of single proteins, most surviving correlations were in kidney cancer. Several pathway predictors that survived the training/test set approach demonstrated marked associations with patient outcome in the overall sample sets ( Supplementary Fig. 12 ). PhosphoSRC (SRCpY416) and the transferrin receptor (TFRC) showed an association in three diseases suggesting particular importance for outcome. However, the effects of the TFRC on patient outcomes were different across diseases suggesting an interaction with lineage-specific events. TFRC expression was associated with a significantly worse prognosis in LUAD and KIRC. These findings have potential implications for clinical targeting using TFRC for targeted delivery of chemotherapy or other agents [45] . Comparing the performance of the optimized cutoff approach with medians, quartiles or tertiles, more often applied in literature, we note that up to 50% of the predictions from the optimized cutoff approach were confirmed using these alternative cutoffs. However, the optimized cutoff approach, combined with a rigorous training and test set evaluation, performed better in 17 out of 21 (81%) cases (as indicated by lower P -values) compared with the use of median, tertiles or quartiles. Network visualization On the basis of the availability of protein data across a large number of samples, we used a probabilistic graphical model approach [46] , [47] without the inclusion of previous knowledge to create an unbiased signalling network ( Fig. 6 , see Methods). We used the relatively large number of samples per tumour lineage to elucidate links in specific cancers and across multiple cancers, inferring networks using tumour lineage-specific samples. Interplay between nodes was quantified using scores from the graphical model analysis (see Methods) that identify links between nodes while controlling for the effects of all other observed nodes. Several expected links were observed across most tumour types, including pMEK with pERK, beta-catenin with E-cadherin and pPKCdelta with pPKCalpha and pPKCbeta , supporting the ability of RPPA analysis to yield high-quality signalling information from TCGA samples. Other expected links were seen in only a subset of tumours such as pAKT with pPRAS40 and pTSC2 (TuberinpT1462), consistent with differential wiring of signalling pathways in different cancers. A number of other links such as MYH11 with RICTOR, cyclinB1 with FOXM1 and pACC with FASN were not expected and warrant further exploration. The interplay between p85 and PTEN is consistent with our demonstration that p85 is a key determinant of PTEN stability [40] , [48] . The negative link between pAKT and PTEN was expected, but the one between p85 and claudin7 in LUSC was not and may be worthy of further exploration. PI3K/AKT signalling does not link clearly to mTOR, which appears to primarily be downstream of MAPK signalling [49] , [50] , [51] . The relatively weak links in the PIK3K/AKT pathway are striking given the degree of antibody representation for this pathway in the RPPA analysis. Key nodes such as CDK1 unexpectedly linked a wide range of protein pathways. Overall, the data suggest that the EGFR receptor family, together with the linked MEK and MAPK pathways, is the dominant determinant of signalling across the cancer lineages in the Pan-Cancer analysis. Using independent data sets in breast cancer, ovarian cancer and endometrial cancer, as well as published research, many of the strongest protein links in the network could be validated ( Supplementary Fig. 13 and Supplementary Table 15 ), supporting the notion that large RPPA-based protein data sets can be used to ‘learn’ networks in an unbiased manner. Figure 6: Unbiased data-driven signalling network. Unbiased signalling network based on a probabilistic graphical model analysis, visualizing all 11 tumour lineages individually. Interplay between nodes was quantified using scores from the graphical model analysis (see Methods) that identify links between nodes whilst controlling for the effects of all other observed nodes. The strength of links is indicated by the thickness of the line while the colour indicates the tumour lineage in which the link was observed; only the strongest links are shown. Nodes in white are related nodes that were highly correlated and therefore merged before network analysis. The adjacent correlated (green) node was then used for network generation. Positive (negative) correlations are indicated with continuous (dotted) lines. A high-resolution image of the network can be found online ( http://bioinformatics.mdanderson.org/main/TCGA/Pancan11/RPPA ). Full size image Cellular biology is effectuated in considerable part by proteins, and, unfortunately neither DNA copy number nor mRNA expression is able to faithfully predict protein level and in particular the post-translational modifications of proteins that are necessary for function ( Fig. 1 , Supplementary Fig. 1 ) [1] , [2] , [3] , [52] , [53] . Hence, evaluation of the functional proteome offers the ability to complement genomic and transcriptomic analysis in projects like the TCGA for identification of biomarkers and elucidation of underlying biological mechanisms both within and across diseases. The availability of high-quality proteomic data across large numbers of samples makes the case more compelling. In sum, a proteomic view of TCGA data yields insights that cannot be acquired through analysis driven solely by genomics or transcriptomics. The high degree of correlation between proteins, including phosphoproteins, in signalling pathways ( Figs 2 , 4 and 6 , TCPA [11] ) supports the applicability of RPPA analysis to TCGA samples. Further, the ability to construct de novo signalling networks ( Fig. 6 ) that capture many known relationships supports the contention that proteomic data derived from the RPPA analysis of TCGA samples can be used to inform system-level analyses of signalling pathways and networks. Full integrative analysis of the DNA, RNA and protein relationships embodied in the several TCGA data sets will require additional analysis, but a number of interesting observations are immediately apparent. Analysis of this large data set demonstrates that, in general, tumour type and subtype are the dominant determinants of protein levels. This observation highlights the risk inherent in disease-specific studies that commonalities, differences and themes that emerge across tumour types will remain undiscovered. We therefore implemented a computational approach, MC, to decrease the dominant effect of tissue-specific protein expression. This approach allowed for the discovery of processes that drive cellular behaviour across tumour types and made it possible to identify tumour characteristics that warrant exploration as therapeutic opportunities. The analysis of individual therapeutically relevant proteins (for example, HER2, Figs 1 and 5 ) and pathways ( Fig. 4 ) permitted classification of patient samples based on pathway activity and therapeutic tractability across different tumour types. The ability of the Pan-Cancer analysis to identify the discordance between HER2 CNV, mRNA expression and protein expression in colorectal and serous endometrial cancers ( Fig. 1 ) argues that a broad protein-based analysis of patient samples across multiple diseases can highlight potential therapeutic opportunities not obvious from studies within single diseases or driven by RNA and DNA analysis alone. The pathway analysis ( Fig. 4 , Supplementary Figs 6–9 ) identifies multiple protein changes that are associated with the same functional outcome (that is, pathway activation) in different samples and tumour types ( Fig. 4 ). A number of proteins and genomic events correlate with pathway scores, developed using proteins defined by literature review ( Fig. 4 , Supplementary Figs 6–9 ). Although some of those relationships could be identified by including members of upstream or downstream signalling or interacting pathways, many of the associations would not be predicted a priori, demonstrating that these approaches offer the potential for discovery of novel pathway connections. The ability to identify unexpected correlations was particularly clear in the network analysis ( Fig. 6 ). For example, the strong links between MYH11 and RICTOR and between ETS1 and pPEA15 across tumour types offer opportunities for discovering new functional relationships. Some associations we reported, such as that of the mTOR pathway with MEK and MAPK, while supported by the literature [49] , [50] , [51] , [54] do not currently receive adequate consideration. Although molecular pathways often seem ‘set in stone’, the identification of unbiased signalling networks using large data sets can provide a powerful tool to identify tissue-specific networks, as well as to demonstrate the importance of ‘non-canonical’ interplay, allowing for re-conceptualization of networks and the role they play in specific diseases. A major goal of the molecular characterization of tumours is the identification of tumour subsets and specific aberrations that can be used in the clinic as biomarkers and/or for targeted therapy (either single-agent or in combination). A bird’s eye view of the functional proteome of large sample sets encompassing multiple tumour lineages may help to suggest potential unexpected targets that are applicable to disease subsets or across diseases. The ability to identify many biomarkers associated with patient outcome (TCPA) and the ability of a set of biomarkers to pass a rigorous training/test set approach ( Supplementary Table 14 ) suggest that additional Pan-Cancer analyses, as well as mechanistic analyses, of the current proteomics study will improve our ability to understand tumorigenesis and identify new markers and targets. Description of the protein data Proteomic data were generated by RPPA across 3,467 patient tumours obtained from TCGA, including 747 breast (BRCA), 464 colon and rectal adenocarcinoma (COAD and READ), 454 renal clear cell carcinoma (KIRC), 412 high-grade serous ovarian cystadenocarcinoma (OVCA), 404 uterine corpus endometrial carcinoma (UCEC), 237 lung adenocarcinoma (LUAD), 212 head and neck squamous cell carcinoma (HNSC), 195 lung squamous cell carcinoma (LUSC), 127 bladder urothelial carcinoma (BLCA) and 215 glioblastoma multiforme (GBM). Those were all the samples we could obtain from TCGA and no samples were excluded. The result is, to our knowledge, the largest and most diversified database of tissue protein levels yet available, an unparalleled basis for rich functional analysis. RPPA methodology has been described in refs 4 , 5 , 6 , 7 , 8 , 9 , 10 and is also provided in the Supplementary Methods . In total, 181 high-quality antibodies targeting total ( n =128), cleaved ( n =1), acetylated ( n =1) and phosphoproteins ( n =51) were used (detailed in Supplementary Data 9 ). In the RPPA assay, antibodies to phosphoHER2 and phosphoEGFR have been noticed to cross-react, especially when the opposite molecule is present at very high levels. This mainly concerns EGFRpY1068 (but not EGFRpY1173), which cross-reacts with overexpressed HER2pY1248. Taking into account their favourable signal:noise ratio (10:1), useful information is contributed by both if expressed differentially, and they are thus both included. The antibodies encompass major functional and signalling pathways of relevance to human cancer. Pathways included are proliferation, DNA damage, polarity, vesicle function, EMT, invasiveness, hormone signalling, apoptosis, immunological, stromal, TGFα/β, transmembrane receptors, metabolism, LKB1/AMPK, TSC/mTOR, PI3K/Akt, Ras/MAPK, Hippo, Notch and Wnt/beta-catenin signalling ( Fig. 6 and Supplementary Fig. 14 ) with minimal redundant information ( Supplementary Fig. 15 ). Supplementary Fig. 16 shows a representative image of a typical antibody slide. The numbers of patient samples and antibodies are greater than those presented in previous TCGA marker papers [4] , [5] , [6] , [7] , [8] , [9] , [10] based on the availability of additional samples as well as validation of additional antibodies. The detailed TCGA data sets are available online ( https://tcga-data.nci.nih.gov/tcga ) and combined with a number of visualization and analytic tools from TCPA ( http://app1.bioinformatics.mdanderson.org/tcpa/_design/basic/index.html ). High-resolution images of all heatmaps and the network are available online ( http://bioinformatics.mdanderson.org/main/TCGA/Pancan11/RPPA ). Some key clinical variables are shown in Supplementary Tables 16,17 ; extensive clinical information for all lineages is available online ( https://tcga-data.nci.nih.gov/tcga ) and available in the various TCGA marker papers [4] , [5] , [6] , [7] , [8] , [9] , [10] . Protein correlations To match the 181 antibodies available, 162 unique mRNAs were selected from downloaded RNASeqV2 data ( https://tcga-data.nci.nih.gov/tcga ), resulting in 184 matched and 24,282 random protein:mRNA pairs. Spearman’s rank correlations were computed on both the random and matched pairs, with associated P -values ( Supplementary Data 1,2 and at http://bioinformatics.mdanderson.org/main/TCGA/Pancan11/RPPA ). The ρ -values of the matched pairs were plotted in histogram form; the ρ -values of the random pairs are represented as a background curve ( Fig. 1a , Supplementary Fig. 1 ). Student’s t -test was used to compare the ρ -values of all matched pairs with the ρ -values of all random pairs (mean matched pairs: 0.3; mean random pairs: −0.006) and showed a significant difference ( P <2.2e−16). For miRNA versus protein, because the number of miRNAs and proteins were small, we computed all pair-wise Spearman’s rank correlations with t -test P -values ( Supplementary Data 3 ). For the CNV versus protein expression analysis, we divided the samples into groups of amplified versus copy-number neutral and deleted versus copy-number neutral, and computed the mean fold changes in protein expression. Similarly, to compare mutation versus protein, we divided the samples into mutated versus wild-type and computed the fold changes in protein expression. We then used t- tests to evaluate statistical significance of the fold changes ( Supplementary Data 5–8 and at http://bioinformatics.mdanderson.org/main/TCGA/Pancan11/RPPA ). Furthermore, we computed all pair-wise protein:protein correlations using the entire Pan-Cancer data set, in total 16,290 correlations ( Supplementary Data 4 and at http://bioinformatics.mdanderson.org/main/TCGA/Pancan11/RPPA ). The top 10% had a Spearman’s rank correlation coefficient magnitude of 0.3 or higher (Bonferroni-adjusted P ≤3.67e−67). Consequently, we considered a correlation magnitude of 0.3 or higher (sign independent) as a reasonable cutoff threshold for the analysis presented in the pathway sections of this study ( Fig. 4 , Supplementary Figs 6–10 , Supplementary Table 13 ). Discriminator selection To detect the discriminating biomarkers for each cluster (obtained by hierarchical clustering using the RPPA data normalized by either RBN or MC), LIMMA [55] was used for the continuous data (protein, mRNA, miRNA) by comparing samples in each cluster with samples in all the other clusters together; information gain [56] was used to select the categorical discriminators (mutation). The resulting data were sorted by decreasing order of the log-odds for the former and by decreasing information gain for the latter method. The top 25 most significant discriminators are shown in Supplementary Tables 2–5 (RBN) and Supplementary Tables 9–12 (MC). The complete overview of protein, mRNA, miRNA and mutation discriminators can be accessed online ( http://bioinformatics.mdanderson.org/main/TCGA/Pancan11/RPPA ). BRCA and UCEC subdivision For BRCA subtypes, first the reactive subtypes were classified according to the method described in the TCGA marker paper [5] . The other subtypes were then classified based on PAM50. For UCEC subtype classification, serous samples were first selected based on the integrative cluster (serous-like) reported in the TCGA marker paper [10] . Clinical histopathological subtype ( https://tcga-data.nci.nih.gov/tcga ) was used in any remaining cases. HER2 cutoffs Normal tissues for the lineages studied in this paper have been reported to have low or medium HER2 levels ( http://www.proteinatlas.org/ENSG00000141736/tissue/staining+overview ) [57] . To identify the threshold of HER2 mRNA and protein expression in breast cancer that could classify tumours as HER2-positive, we obtained PAM50 classifications for all the TCGA breast cancer samples and divided them into two groups; HER2-positive and nonHER2-positive samples. We used the conjunctive rule algorithm in Weka software [58] to determine the best HER2 total protein cutoff that separated the HER2-positive from the nonHER2-positive samples based on HER2 ( ERBB2 ) copy number. The best protein threshold was found to be 1.46, which yielded 93% accuracy of prediction and a receiver operator characteristic (ROC) area under the curve (AUC) of 0.81. We did a similar analysis using HER2 mRNA and found a best cutoff of 14.26 (in log 2 frame), which yielded an accuracy of 93% and a ROC AUC of 0.82. In addition to trastuzumab, other drugs targeting HER2 have entered clinical trials, such as TDM1, for which HER2 expression on the cell surface is sufficient to achieve preferential binding to the cell and therapeutic impact. Since data for TDM1 response are not readily available, a threshold of HER2 expression that may be sufficient to expect a response could not be calculated. We therefore compared samples in which HER2 was amplified versus not amplified, aiming to find a threshold that might be reasonable to test. Using the dot plots, a protein threshold of ≥1.00 was adopted, approximately equivalent to 3+ on immunohistochemistry of clinical samples in breast cancer. The crosstab in Fig. 1b gives the breakdown of percentage of samples above these thresholds for each tumour. If a tumour lineage had more than 10% HER2-positive samples according to any of the cutoffs, this is indicated in red. General heatmap section A two-way unsupervised hierarchical clustering analysis was used to discover the groups of biological objects sharing common characteristics [59] , [60] , and a two-dimensional heat map was drawn to visualize protein expression patterns. We used Ward linkage as the agglomeration rule and 1-Pearson correlation as the dissimilarity metric. On the basis of protein expression patterns and guided by the clustering dendrogram, we divided the RBN data set into eight clusters and the MC dendrogram into seven clusters. As seen in the RBN heatmap, most clusters represented one major disease. Exceptions were clusters_E and _F. On the basis of the recent TCGA marker paper [5] , the hormone-responsive breast cancer cluster (cluster_A) in the RBN dendrogram was further divided into two subclusters, A1 (reactive breast cancers) and A2 (remaining luminal breast cancers). On the basis of marked enrichment with clinically relevant proteins, cluster_II in the MC dendrogram was further divided into two subclusters, cluster_IIa (HER2 elevated) and cluster_IIb (EGFR elevated). Hierarchical clustering analysis was performed using R, version 2.15.1 ( http://www.r-project.org/ ). Heatmaps were generated using an NGCHM R-package [59] . Annotation bars were added to the heatmap that included tumour lineage, purity and ploidy; stromal and immune scores; BLCA subtype and PAM50 classification (BRCA). Significantly mutated genes (present in more than 5% of tumours in the data set, resulting in 16 genes) are included as are the two most frequently observed amplifications. Statistical significance for the annotation bars on top of the various heatmaps was calculated by χ 2 -test (tumour lineage, mutations and amplifications), ANOVA’s F test (purity, ploidy stromal and immune score) and Fisher’s exact test (PAM50 and BLCA subtypes). Data are missing for BLCA subtype (15/127), BRCA subtype (52/747) and HER2 and MYC amplification (64/3,467). Batch effects removal The 3,467 RPPA Pan-Cancer samples were run in six batches in total, resulting in potential batch effects on merging the sets. Batch effects in RPPA data are a known concern, even when controlling for critical materials such as the treated glass slides, antibodies, enzymes and suppliers [62] . A new algorithm, replicates-based normalization (RBN), was therefore developed, using replicate samples run across multiple batches to adjust the data for batch effects. The underlying hypothesis is that any observed variation between replicates in different batches is primarily due to linear batch effects plus a component due to random noise. Given a sufficiently large number of replicates, the random noise is expected to cancel out (mean=zero by definition). Remaining differences are treated as systematic batch effects. We can compute those effects for each antibody and subtract them out. In one batch, many samples with duplicates in the other five batches were run and could therefore serve as anchor for all batches. The number of duplicate samples with each batch varied between 71 and 207. This batch was designated ‘anchor’ batch and was used unchanged. We then computed the means and s.d. values of the common samples in the anchor batch and each of the other batches. The difference between the means of each antibody in the two batches and the ratio of the s.d. values provided an estimate of the systematic effects between the batches for that antibody (both location-wise and scale-wise). Each data point in the non-anchor batch was adjusted by subtracting the difference in means and multiplying by the inverse ratio of the s.d. values to cancel out those systematic differences. Whether RBN could successfully integrate batches, while preserving known biological variation, was tested on TCGA breast cancer samples. As breast cancer subtypes (luminal, HER2 -positive and basal-like) are well established [13] , we expected the subtypes from different batches to cluster together. Without RBN, the batches clustered by batch. After RBN, the batches clustered by subtypes spanning multiple batches ( Fig. 2 ). Details of these experiments have been published previously [63] . Reducing tissue differences to cluster across tumours Using RBN, batches of RPPA data could be merged successfully. However, as protein levels of different tumours are (usually) quite distinct from each other, most samples clustered by tumour lineage ( Fig. 2 ). Normal cells differentiate into different tissues by turning on or off different sets of genes. When cells become malignant, they retain many tissue-specific expression characteristics. We hypothesized that tissue-specific effects exist because of those expression differences and equalizing the median expression of genes across tumours might reduce those effects. A gene that is turned off in all the samples of a tumour lineage will have little variation in expression, similar to a gene that is always turned on, which will also have little variation, but an overall high level. To compare across tumour lineages, we started with the batch-corrected RBN data and took sets of all samples belonging to each tumour lineage. We subtracted the median protein expression across all the samples from a single lineage (median centering, MC), making the median expression of all proteins within any given tumour equal to zero. That removed the fixed, bias component from that tissue lineage but retained the variable component found in each tumour. Since the tissue-specific component had been removed, we could then compare the variable component (which was relative in scale) in each tumour sample across different tissues. That allowed for the comparison between samples with high/low expression in one tumour and samples with high/low expression in another tumour, such as HER2 or EGFR expression. Basal-like breast cancer was treated as a separate tumour lineage from the other breast cancer samples due to its expression profile being so different that it did not merge with any other tumour or even other breast samples during RBN clustering. Tumour purity and ploidy We obtained tumour purity and ploidy data based on the ABSOLUTE algorithm [64] from TCGA Pan-Cancer working group. We calculated stromal and immune scores based on the ESTIMATE algorithm using the TCGA Pan-Cancer gene expression data set (syn1695373, https://www.synapse.org/#!Synapse:syn1695373 (ref. 65 )). Pathway analysis For each pathway, members, illustrated in Supplementary Table 13 , were predefined based on a Pubmed literature search on review articles describing the various pathways in detail. RBN RPPA data were median-centred and normalized by s.d. across all samples for each component to obtain the relative protein level. The pathway score is then the sum of the relative protein level of all positive regulatory components minus that of negative regulatory components in a particular pathway. We averaged antibodies targeting different phosphorylated forms of the same protein with ρ >0.85 (Pearson’s correlation). The pathway scores are visualized in the bar just above the heatmap and as a dotplot below the heatmap (median and inter-quartile range indicated, Fig. 4c–f , Supplementary Figs 6–9 ). Subsequently, for each version of the pathway scores (RBN or MC derived), a Spearman’s rank correlation test was performed between each pathway score and every protein. If the ρ was >0.3 or <−0.3, the protein was included in the heatmap. Regardless of the ρ , pathway members for the given pathways were included. Annotation bars (from Fig. 2 ) were included if they were statistically significantly associated with the pathway ( P <0.05, Kruskal–Wallis test, n =3,467), corrected for multiple testing [66] . Tumour lineage and cluster were included to facilitate interpretation. For each pathway heatmap (RBN or MC), the samples were first sorted by the alphabetic order of either cluster or tumour, and then by the increasing order of a pathway score. Using the heatmap method described above, two additional summary heat maps for the pathway scores (RBN and MC) were generated ( Fig. 4a,b ) to provide an overall view of the relationships between tumours, unsupervised clusters and pathways. Mean pathway scores were calculated for each tumour as well as cluster variables, and the combined mean pathway scores were standardized for each pathway across all tumour and clusters. In both the individual pathway plots and the heatmap summary plots, hierarchical clustering was based on Pearson’s correlation-based distance matrices [67] and Ward linkage. The dynamic heat maps were generated using the R-package NGCHM [61] . Each cell in the heatmap represents the mean pathway score of all the samples in that cluster or tumour lineage, with blue representing a suppressed pathway, red representing an activated pathway and white representing neither. Supplementary Fig. 10a,b shows a similar measure of pathway activity, but on the absolute scale. The Supplementary Figure is derived as follows. First, the RPPA data set (either RBN or MC normalized) is globally scaled so that the protein expression level measurements have zero mean and unit s.d. over all samples. Next, for each cluster and tumour lineage, we calculate the mean (scaled) protein expression level for each protein. We then convert these means to their absolute value (as low or high mean protein levels could both be markers of pathway activity), obtaining an absolute mean protein level for each protein in each cluster or tumour lineage. Finally, for each pathway, we calculate the average of the absolute mean levels over the proteins that participate in the pathway. This value is designated the differential pathway activity score, as it indicates the deviation from the mean expression of a pathway in a given cluster or tumour lineage, and can thus be seen as a proxy for pathway activation/deactivation. Actionable protein analysis The analysis focused on the potential ability of proteomics to predict response to proteins currently of increased interest, due to proposed targetability or potentiality as a drug target in the drug development stage. The list of proteins is not exhaustive, but rather includes many different processes and pathways with varying importance in different tumour lineages included in this study. In the Supplementary Methods , registered trials targeting many of these proteins are included. To visualize the expression pattern of these 25 proteins, heatmaps were generated [61] using the RBN data set ( Fig. 5 ). Proteins were ordered by unsupervised hierarchical clustering and samples were ordered by cluster (disease) membership and within each, ordered by unsupervised hierarchical clustering. Ward’s method and 1-Pearson correlation were used as a dissimilarity metric and linkage. Network analysis Networks were estimated using statistical models known as a probabilistic graphical models (specifically Gaussian graphical models) [47] . These models use an undirected graph or network to describe probabilistic relationships between variables. In contrast to pair-wise correlation analysis, the networks are rooted in a global, multi-dimensional approach that identifies links between nodes while controlling for the effects of all other observed nodes. Statistical inference of networks is a so-called ‘high-dimensional’ problem because network descriptions require a large number of parameters relative to available sample sizes (especially at the disease or cluster level). This motivates a need for regularization to learn sparse, parsimonious networks and thereby control over-fitting. We used l 1 -penalization for this purpose, specifically via an algorithm known as graphical lasso [46] , as implemented in the R-package huge [68] . A parameter λ that controls the strength of penalization was set by 10-fold cross-validation in all cases. To prevent artefacts that can arise due to duplicated nodes, related nodes that were relatively highly correlated were merged before network analysis. In each such case, only one of the set of correlated nodes was used for network inference and the remaining merged nodes are shown in white. Since protein levels are measured in arbitrary units (depending on affinity and avidity of specific antibodies), for each network the data were standardized before applying the graphical lasso, such that each protein had zero mean and unit variance. Outcome analysis A training test approach was adopted for survival analysis. In each of the 11 tumour lineages, samples with survival data available were randomly divided into training (2/3) and test (1/3) sets with balanced events in both sets. The training set was used to obtain an optimized cutoff, which was ‘locked’ (that is, used without change) on the test set. Essentially, samples were sorted based on the protein expression of the interesting gene or pathway score. Each possible cutoff in the middle 60% of samples was checked using a Cox’s regression model. The cutoff with lowest P -value was chosen as the optimized cutoff. In the test set, samples were divided into high and low groups according to this optimized cutoff by either percentage or absolute value. Then the hazard ratio, Wald’s test P -value and Kaplan–Meier survival curves of the two groups were examined by Cox’s regression analysis. Only the predictors that were successfully validated in the test set are shown in Supplementary Table 14 . Kaplan–Meier survival curves were generated to illustrate the survival differences in the four significant pathways using the whole sample set ( Supplementary Fig. 12 ). How to cite this article: Akbani, R. et al. A pan-cancer proteomic perspective on The Cancer Genome Atlas. Nat. Commun. 5:3887 doi: 10.1038/ncomms4887 (2014).